Stabilizing short-lived Schiff base derivatives of 5-aminouracils that activate mucosal-associated invariant T cells Mucosal-associated invariant T (MAIT) cells are activated by unstable antigens formed by reactions of 5-amino-6- D -ribitylaminouracil (a vitamin B2 biosynthetic intermediate) with glycolysis metabolites such as methylglyoxal. Here we show superior preparations of antigens in dimethylsulfoxide, avoiding their rapid decomposition in water ( t 1/2 1.5 h, 37 °C). Antigen solution structures, MAIT cell activation potencies (EC 50 3–500 pM), and chemical stabilities are described. Computer analyses of antigen structures reveal stereochemical and energetic influences on MAIT cell activation, enabling design of a water stable synthetic antigen (EC 50 2 nM). Like native antigens, this antigen preparation induces MR1 refolding and upregulates surface expression of human MR1, forms MR1 tetramers that detect MAIT cells in human PBMCs, and stimulates cytokine expression (IFNγ, TNF) by human MAIT cells. These antigens also induce MAIT cell accumulation in mouse lungs after administration with a co-stimulant. These chemical and immunological findings provide new insights into antigen properties and MAIT cell activation. T cells use their surface T-cell receptors (TCRs) to recognize specific microbial antigens that are captured and presented by antigen-presenting cells (APC). T cells are typically activated by peptides [1] or lipids [2] , [3] , but mucosal-associated invariant T cells (MAIT cells) [4] are innate-like T cells in the blood [5] , [6] , liver [7] , [8] , [9] , [10] , [11] , [12] and gut mucosa [9] , [13] , [14] that are activated instead through covalent binding to pyrimidine derivatives that feature a chemically unstable α-iminocarbonyl Schiff base component (R 1 CO–CR 2 =NH–) [15] , [16] . These antigens are formed from 5-amino-6- D -ribitylaminouracil ( 1 , 5-A-RU), a key intermediate in the biosynthesis of riboflavin (vitamin B2) by many bacteria and fungi [15] , [17] . During microbial riboflavin biosynthesis, this intermediate undergoes enzyme-catalyzed condensation with 3,4-dihydroxy-2-butanone-4-phosphate ( 2 ), followed by rapid cyclization to form 6,7-dimethyl-8-( D -ribityl)lumazine ( 4a ), which subsequently dismutates to give riboflavin ( Fig. 1a ). However, 1 can also react through non-enzymatic Schiff base condensation with α-dicarbonyl compounds ( 5a-c ) ( Fig. 1a ), such as glyoxal ( 5b ) and methylglyoxal (pyruvaldehyde, 5c ) [18] , [19] , derived from mammalian glycolysis or bacterial metabolism to give the adducts 5-(1-methyl-2-oxopropylideneamino)-6- D -ribitylaminouracil (5-MOP-RU, 3a ; a riboflavin biosynthetic intermediate), 5-(2-oxoethylideneamino)-6- D -ribitylaminouracil (5-OE-RU, 3b ), and 5-(2-oxopropylideneamino)-6- D -ribitylaminouracil (5-OP-RU, 3c ). 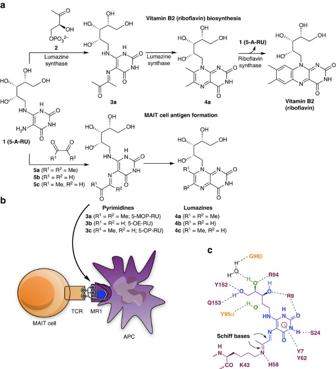Figure 1: Glycolysis metabolites react with a vitamin B2 biosynthetic intermediate to create MAIT cell antigens. (a) Enzymatic biosynthesis of vitamin B2 (top), and formation of antigens from biosynthetic intermediate1by condensation with glycolysis metabolites5a-c(bottom). (b) Complex of antigen (blue) sandwiched between MR1 (purple) on the surface of an antigen-presenting cell APC and T-cell receptor protein TCR (orange) on the surface of a MAIT cell. (c) Interactions observed in a ternary crystal structure of a human MAIT TCR-3c-MR1 complex15, showing antigen (blue)···MR1 (purple) and antigen (green)···TCR (orange) contacts, with an extended conjugated system involved inπ-interactions (dashed circle). Figure 1: Glycolysis metabolites react with a vitamin B2 biosynthetic intermediate to create MAIT cell antigens. ( a ) Enzymatic biosynthesis of vitamin B2 (top), and formation of antigens from biosynthetic intermediate 1 by condensation with glycolysis metabolites 5a-c (bottom). ( b ) Complex of antigen (blue) sandwiched between MR1 (purple) on the surface of an antigen-presenting cell APC and T-cell receptor protein TCR (orange) on the surface of a MAIT cell. ( c ) Interactions observed in a ternary crystal structure of a human MAIT TCR- 3c -MR1 complex [15] , showing antigen (blue)···MR1 (purple) and antigen (green)···TCR (orange) contacts, with an extended conjugated system involved in π -interactions (dashed circle). Full size image These α-iminocarbonyl adducts 3a-c are very unstable chemical entities, susceptible to hydrolysis or intramolecular cyclization to give bicyclic lumazines 4a-c . Nevertheless, 3b and 3c persist long enough to be captured and stabilized through a covalent bond with Lys43 of the major histocompatibility complex (MHC) class I-related protein (MR1) [15] . This creates a second Schiff base and anchors 3b-c to MR1 for subsequent presentation to the TCR of MAIT cells ( Fig. 1b ). The formation of this covalent bond between the antigen and the antigen-presenting protein is a striking and novel way to stabilize a T-cell antigen. Furthermore, although a Schiff base ligand-protein covalent bond is not without precedence in nature (for example, pyridoxal phosphate, fructose 1,6-bisphosphate, retinal) [20] , the linkage between the uracil and MR1 involves two consecutive Schiff bases, creating a 1,2-diimino moiety (–NH=CR 1 –CR 2 =N–; Fig. 1c ) that is unprecedented in biological chemistry. Crystal structures of the MR1-antigen-TCR ternary complexes reveal that the antigen is almost encircled by MR1, with multiple hydrogen bonds from the uracil and ribityl components to MR1 and TCR residues ( Fig. 1c ) [15] , [21] , [22] , [23] , [24] . Two tyrosine residues from MR1 (Y7, Y62) are positioned for π -interactions with the pyrimidine ring. The novelty and potential immunological importance of these structures demands an understanding of the synthesis, structure, and chemical properties of 3a-c , as well as the identification of stereochemical requirements for antigen potency and stability and for MR1-dependent MAIT cell activation, all of which are described here. Synthesis of unstable MAIT cell antigens The condensation of uracil derivative 1 with α-dicarbonyls 5 in water is known [25] , [26] , [27] , [28] , [29] , [30] , [31] to produce lumazines ( Fig. 1a ), but the anticipated putative imine intermediates 3a-c had not been isolated nor characterized prior to our work. These fleeting intermediates cannot be efficiently synthesized in water for biological applications for three reasons. First, the condensation of diamine 1 with unsymmetrical α-dicarbonyls 5 generates a mixture of inseparable regioisomers. Second, formation of imines (as in 3a-c ) and their hydrolyses are reversible in water. Third, 3a-c undergo rapid intramolecular condensation between amine and carbonyl groups to form bicyclic lumazines 4a-d ( Fig. 1a ), a process likely to be driven thermodynamically by aromatization. These limitations were evident when the reactions between 1 and 5a-c were monitored in water ( Fig. 2 ). For example, the reaction with 5c was monitored at different pH (pH 7.4, PBS; pH 5.4, 20 mM NH 4 OAc buffer, 150 mM NaCl) and temperature (37 and 15 °C) using analytical LCMS ( Supplementary Fig. 1 ). Regioisomers can form depending on whether the C-5 amine of 1 condenses with the more reactive aldehyde or the ketone of 5c to give 4c or 4d , respectively (see Supplementary Figs 22–30 for NMR spectra). The rate of formation of imines 3c-d and their subsequent cyclization to lumazines 4c-d were highly dependent on reaction conditions, with 4c forming preferentially over 4d with increasing acidity or temperature ( Supplementary Fig. 2 ). The concentration of 3c typically peaked at approximately 5–10 min ( Supplementary Fig. 1 ). Compound 1 reacted even faster with 5b than 5c , with the concentration of 3b peaking at 1 min before completely cyclizing within 30 min (pH 7.4, PBS; 15 °C) to 4b ( Supplementary Fig. 3 ). 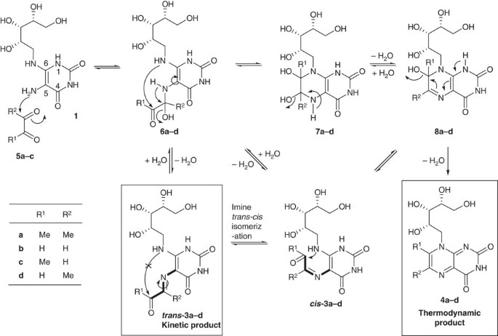Figure 2: Proposed mechanism for reaction between 1 and 5 to produce uracil and lumazine derivatives. These reactions are reversible in water, but dehydrative cyclization drives formation of thermodynamically more stable aromatic lumazine derivatives4. Polar aprotic solvents may facilitate kinetic control of these equilibria and enabletrans-3to persist in solution. Figure 2: Proposed mechanism for reaction between 1 and 5 to produce uracil and lumazine derivatives. These reactions are reversible in water, but dehydrative cyclization drives formation of thermodynamically more stable aromatic lumazine derivatives 4 . Polar aprotic solvents may facilitate kinetic control of these equilibria and enable trans - 3 to persist in solution. Full size image We discovered that the unstable intermediates 3a-c could be isolated as kinetic products by exploiting key stereochemical properties, as revealed by the reaction mechanism between 1 and 5 ( Fig. 2 ). Diamine 1 should react with dicarbonyl 5 to preferentially form hemiaminal 6 , as the C-5 amine is more nucleophilic than the C-6 amine at the β-position of a vinylogous amide ( Supplementary Fig. 2 ). Elimination of water from 6 gives trans - 3 , in which the amine and carbonyl groups are held apart by the trans -configuration to prevent cyclization, unlike cis - 3 , which is preorganized for cyclzation. If the reaction of 1 and 5 was carried out in water, the reaction proceeds under thermodynamic control, with trans - 3 rehydrating to 6 followed by bond rotation and cyclization via 7 (or cis - 3 ) and 8 to give lumazine 4 ( Fig. 2 ). However, the reaction between 1 and 5 in a non-aqueous solvent should proceed under kinetic control. In this scenario, trans - 3 should form faster than cis - 3 from 6 for steric reasons ( Supplementary Fig. 4 ). Once formed, trans - 3 is unlikely to isomerize to cis - 3 as this transformation has a large and prohibitive activation energy barrier [32] , estimated by ab initio gas phase density functional theory (DFT) calculations to be 20–28 kcal mol −1 ( Supplementary Fig. 5 ). Thus, if the formation of trans - 3 from 6 was also faster than the formation of 7 , then trans - 3 should accumulate as the kinetic product ( Fig. 2 ). The choice of solvent can significantly alter the outcome of a chemical reaction and dictate whether it is kinetically or thermodynamically controlled [33] , [34] , [35] . In order to obtain the kinetic product trans - 3 , the condensation of 5c with model compound 5-amino-6-methylaminouracil (an analogue of 1 ) was investigated by NMR spectroscopy in a polar aprotic solvent (nitromethane- d 3 , DMF- d 7 or DMSO- d 6 ). However, imine formation without simultaneous cyclization was only observed in DMSO- d 6 ( Fig. 3a ), consistent with it having the largest dielectric constant and an ability to accept hydrogen bond donors. These properties respectively accelerate the cationic E1 dehydration over the cyclization reaction, and suppress imine rehydration through solvation of liberated water molecules by DMSO ( Supplementary Fig. 6 ). The reactions between 1 and 5a-c in anhydrous DMSO- d 6 were studied by 1 H and 13 C NMR spectroscopy ( Fig. 3 ). Formation of 3a-c was observed clearly within 1 h (for example, Fig. 3b ). The reaction of 1 with the unsymmetrical 5c gave the regioisomer 3c exclusively, consistent with the greater reactivity of the formyl than the acetyl group in 5c ( Fig. 3a ). 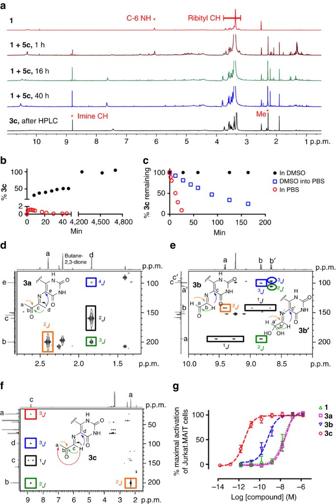Figure 3: Formation and solution structures of uracil-based antigens that activate MAIT cells. (a) Exclusive formation of 5-OP-RU3cfrom1and5cin DMSO-d6, as monitored by1H NMR spectroscopy, with the characteristic signals of1and 5-OP-RU3cas indicated. (b) Formation of 5-OP-RU3cin DMSO (black) versus PBS buffer (red). In PBS buffer (red, 2.62 mM of1, 7.86 mM of5c, pH 7.4, 37 °C),3creached a maximum concentration corresponding to only 1.1% conversion of1at 5 min. In DMSO (black, 31.8 mM1and 34.5 mM5c, room temperature), 5-OP-RU3creached 100% conversion after 2 days and then plateaued. (c) Stability of 5-OP-RU3cin DMSO (black), PBS buffer (red) and after the DMSO solution was diluted into PBS buffer (blue). Data for PBS buffer were extracted fromb(red) at the time the maximum 5-OP-RU3cconcentration was reached (that is, 5 min after mixing). (d–f) HMBC NMR spectra of3a-c(DMSO-d6), respectively. Square boxes indicate correlations for the aldehyde form of3b, and circles for its hydrate form3b′. Arrows and boxes indicate key1H–13C long-range correlations that unambiguously characterize the compounds.Jrefers to heteronuclear coupling through 1, 2, 3 or 4 bonds. (g) MAIT cell activation. Data represent mean±s.e.m. (n=3). The α-dicarbonyls5a-c, lumazines4a-band the solvent DMSO-d6were inactive (up to 15 μM), while4cand4dhad only very weak activity at the highest concentrations tested (EC50>100 nM). Figure 3: Formation and solution structures of uracil-based antigens that activate MAIT cells. ( a ) Exclusive formation of 5-OP-RU 3c from 1 and 5c in DMSO- d 6 , as monitored by 1 H NMR spectroscopy, with the characteristic signals of 1 and 5-OP-RU 3c as indicated. ( b ) Formation of 5-OP-RU 3c in DMSO (black) versus PBS buffer (red). In PBS buffer (red, 2.62 mM of 1 , 7.86 mM of 5c , pH 7.4, 37 °C), 3c reached a maximum concentration corresponding to only 1.1% conversion of 1 at 5 min. In DMSO (black, 31.8 mM 1 and 34.5 mM 5c , room temperature), 5-OP-RU 3c reached 100% conversion after 2 days and then plateaued. ( c ) Stability of 5-OP-RU 3c in DMSO (black), PBS buffer (red) and after the DMSO solution was diluted into PBS buffer (blue). Data for PBS buffer were extracted from b (red) at the time the maximum 5-OP-RU 3c concentration was reached (that is, 5 min after mixing). ( d – f ) HMBC NMR spectra of 3a-c (DMSO- d 6 ), respectively. Square boxes indicate correlations for the aldehyde form of 3b , and circles for its hydrate form 3b′ . Arrows and boxes indicate key 1 H– 13 C long-range correlations that unambiguously characterize the compounds. J refers to heteronuclear coupling through 1, 2, 3 or 4 bonds. ( g ) MAIT cell activation. Data represent mean±s.e.m. ( n =3). The α-dicarbonyls 5a-c , lumazines 4a-b and the solvent DMSO- d 6 were inactive (up to 15 μM), while 4c and 4d had only very weak activity at the highest concentrations tested (EC 50 >100 nM). Full size image Imines 3a-c were much more stable in DMSO than in water ( Fig. 3c and Supplementary Fig. 9 ), remaining essentially unchanged (>90%) after 2 days in DMSO- d 6 at 22 °C. Thus, by using a common aprotic solvent, the outcome of the reaction was completely diverted to a single kinetic end point without the use of protecting groups, overcoming the substantial challenge posed by the instability of 3a-c in water where they convert rapidly to lumazines 4a-c (ref. 36 ). After extensive optimization of conditions, imine 3c could even be purified by rpHPLC by minimizing its exposure to water and acid ( Fig. 3a and Methods). However, 3a and 3b were much less stable in aqueous media and could not be further purified. Imines 3a-c were characterized in DMSO- d 6 by 1D and 2D NMR and HRMS ( Fig. 3d–f ; Supplementary Information ). The imines 3a and 3c were single, stable species in DMSO. The reaction between 1 and 5b gave an inseparable mixture of imine 3b , its formyl hydrate ( gem diol) and the symmetrical bis -imine adduct (as characterized by the imine singlet at δ 9.24 p.p.m. and ESI-MS m/z =575 [M+H] + ) in a ratio of 1:1:1.3. Imine 3b showed characteristic coupling ( 3 J HH =8.0 Hz) between the formyl (9.42 p.p.m.) and imine (8.82 p.p.m.) protons. Meanwhile, its hydrate showed a doublet ( 3 J HH =6.7 Hz) with a chemical shift (δ 5.40 p.p.m.) typical for an acetal proton. All three imines 3a-c were single geometric isomers, unambiguously characterized by Heteronuclear Multiple Bond Correlation (HMBC) NMR spectra, indicating key connectivities within and between the α-iminocarbonyl unit and the uracil ring ( Fig. 3d–f ). In 3b and 3c , the imine protons (δ 8.81 and 8.70 p.p.m., respectively) showed 3 J HC correlations to the ring C-5, with the methyl signal at δ 1.82 p.p.m. making the analogous 4 J HC correlation for imine 3a . The imine protons of 3b and 3c also showed 2 J CH correlations to carbonyl carbons ( δ 194.5 and 200.2 p.p.m., respectively), while the methyl proton signal at δ 1.85 p.p.m. of 3a showed a 3 J HC correlation with a carbonyl carbon at δ 199.7 p.p.m., proving that cyclization of 3a-c had not occurred. The chemical stabilities of 3a-c were determined in various aqueous buffers ( Supplementary Fig. 7 ). In PBS buffer (pH 8.0, 15 °C), the half-life of 3a could not be measured as it had completely degraded in <5 min, while 3b decayed exponentially with a half-life of 18 min. The homologue 3c was more stable with a half-life of 14 h, consistent with a slower attack on the more hindered carbonyl of 6c than 6b . The half-life of 3c decreased substantially with increasing acidity and temperature. At 15 °C and 0.065 mM, its half-life decreased to 12 h at pH 6.8 (MilliQ water) to 44 min at pH 5.4. It decayed linearly with time at pH 6.8 and pH 8.0, but exponentially at pH 5.4. Under physiological conditions (PBS, pH 7.4, 37 °C), its half-life was 88 min. In aqueous media, 3c degraded to give exclusively lumazine 4c without forming isomer 4d at pH 6.8–8.0. Next, we evaluated how the 5-OP-RU 3c formation and degradation kinetics impacted on its preparation and potential use as an immunological reagent. In our previous studies, 5-OP-RU 3c was prepared by mixing 5-A-RU 1 with methylglyoxal 5c in aqueous media and then used in immunological studies in vitro . However, when 5-A-RU 1 and methylglyoxal 5c are mixed in PBS buffer (pH 7.4 and 37 °C), 5-OP-RU 3c reaches a maximum conversion of only 1.1%, before very rapidly degrading with a half-life of 12 min, indicating that the purity of the desired compound generated in the mixture was extremely low ( Fig. 3b ). In contrast, when 5-A-RU 1 and methylglyoxal 5c were combined under argon in DMSO- d 6 , 5-OP-RU 3c was formed as the sole product and still intact after 72 h ( Fig. 3a,b ). Prepared in this way, 5-OP-RU 3c was stable in DMSO solution (>95%) for days at room temperature. When this DMSO solution of 5-OP-RU 3c was diluted into aqueous buffer (PBS, pH 7.4, 37 °C) its half-life also increased more than sevenfold (half-life=88 min) ( Fig. 3c ). Thus, pre-forming 5-OP-RU 3c in DMSO- d 6 as a kinetic product and then diluting into aqueous buffer yielded a product of substantially higher purity, in greater quantity and with much higher stability than in our previously reported aqueous preparations. Comparison of MAIT cell activation by 3a-c MAIT activation was evaluated using a well established reporter assay [17] by co-culturing two cell lines (human MAIT TCR-transduced Jurkat T cells and MR1-overexpressed C1R cells, Fig. 3g ). Imine 3c (effector concentration for half-maximum response (EC 50 ) 1.6 pM) was the most potent antigen. Although the high-resolution ternary MR1-antigen-TCR crystal structures of 3b-c were nearly identical [15] , 3b (EC 50 510 pM) was 2 orders of magnitude less potent than 3c , consistent with its reduced chemical stability in water. Imine 3a might also be expected to act as an antigen for the MAIT cell mediated detection of microbial infections due to its structural homology to 3b-c and its role as a putative intermediate in bacterial riboflavin biosynthesis. However, consistent with the inability of mixtures of 1 and 5a to refold MR1 (ref. 15 ), imine 3a (EC 50 24 nM) was found to be significantly less active than 3b-c ( Fig. 3g ), a result attributable to its extreme instability in water. Conformational analysis of 3a-c To better understand the relative potencies and stabilities of 3a-c , which have almost identical chemical structures, ab initio DFT calculations (at the level of B3LYP/6-311+g(d,p)) were used to predict their optimized structures ( Fig. 4a ). Compounds 3b-c showed little deviation from conformations that we observed in crystal structures, with the C-6 nitrogens, uracil rings and iminocarbonyl moieties notably coplanar. This implied that the solution conformations of 3b-c were likely to be close to their optimal MR1-binding conformation, consistent with MR1 requiring 3b-c in order to fold into a biologically functional ternary structure, a process that caused little conformational perturbation to the antigens, according to these calculations. 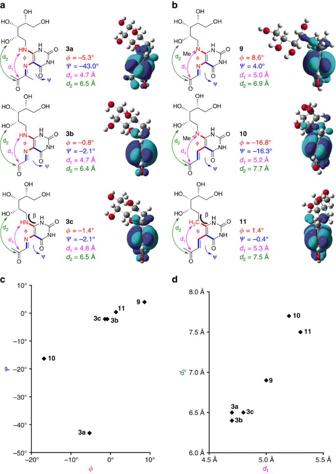Figure 4: DFT optimized conformations of 3a-c and analogues 9–11. (a) Optimized conformers of3a–cand (b) optimized conformers of9–11, which are analogues of3c. Dihedral angles (red) andψ(blue) define the angles formed by 5,6-substituents centred at uracil C5-C6 and 5-substituent to uracil C5-C4, respectively. In order to visualize the twisting of these substituents, the LUMOs (with orbital phases in cyan and blue) are shown for clarity. The incorporation of a methyl group to3c(that is,3a,9or10) resulted in a twisting of the C-5 substituent relative to the ring and an inversion of the LUMO phase at the carbonyl carbon (3aand10). These changes likely impact the ability of the ligands to form non-covalent interactions with MR1 and MAIT TCR (Fig. 1), as well as their reactivity towards the formation of Schiff base with K43 of MR1. (c,d) Plots illustrating the structural similarity of the compounds based on the dihedral angles (red) andψ(blue), and the distancesd1(purple) andd2(green). Figure 4: DFT optimized conformations of 3a-c and analogues 9–11. ( a ) Optimized conformers of 3a – c and ( b ) optimized conformers of 9 – 11 , which are analogues of 3c . Dihedral angles (red) and ψ (blue) define the angles formed by 5,6-substituents centred at uracil C5-C6 and 5-substituent to uracil C5-C4, respectively. In order to visualize the twisting of these substituents, the LUMOs (with orbital phases in cyan and blue) are shown for clarity. The incorporation of a methyl group to 3c (that is, 3a , 9 or 10 ) resulted in a twisting of the C-5 substituent relative to the ring and an inversion of the LUMO phase at the carbonyl carbon ( 3a and 10 ). These changes likely impact the ability of the ligands to form non-covalent interactions with MR1 and MAIT TCR ( Fig. 1 ), as well as their reactivity towards the formation of Schiff base with K43 of MR1. ( c , d ) Plots illustrating the structural similarity of the compounds based on the dihedral angles (red) and ψ (blue), and the distances d 1 (purple) and d 2 (green). Full size image Unexpectedly, 3a had a significantly different modelled conformation to 3b-c despite their structural similarity. Due to a steric clash between the imine methyl and the C-4 uracil carbonyl, the iminocarbonyl and the ribityl moieties were twisted out of the uracil ring conjugation plane by −43.0° ( ψ ) and −5.3° (), respectively. Further, as the imine was twisted out of the plane of ring conjugation, the imine hydration of 3a (to give 6a , Fig. 2a ) would not disrupt conjugation and was likely to incur a lower energetic penalty than 3b-c , leading to increased susceptibility to cyclization and imine hydrolysis. The significantly different electronic structures (based on LUMOs) of 3a and 3b-c were consistent with a loss of conjugation in 3a ( Supplementary Fig. 8 ). Together, the inability to adopt the flat conformation needed for binding and the increased imine hydration susceptibility rationalizes the greatly reduced antigenic activity of 3a relative to 3b-c and represents a crucial distinction between the productive riboflavin biosynthetic intermediate 3a and off-pathway by-products of the much more potent antigens 3b and 3c . The apparent MAIT activity of 3a should therefore be cautiously interpreted, but may be attributable to facile hydrolysis to 1 . Under the cell assay conditions, compound 1 can subsequently react with endogenous 5b-c to give trace 3b-c . Moreover, the potency of 1 , which can neither refold nor form a Schiff base with MR1, was dependent on the concentration of dicarbonyl 5b-c, suggesting that its apparent EC 50 18 nM was also due to its ability to reform trace amounts of 3b-c . Design and synthesis of a stable T-cell antigen Having synthesized the unstable but potent antigens 3b-c , we sought to create a potent antigen that was chemically stable. As the energy-minimized conformations of 3b-c were similar to those found in their ternary TCR-antigen-MR1 crystal structures [15] ( Fig. 4a ), we hypothesized that MAIT cell activation may be related to conformational similarity of an antigen to 3c in the crystal structure. Thus, analogue 9 was designed from 3c , in which the nucleophilic C-6 amine was N -methylated in order to retard cyclization ( Fig. 4b ). Then, 10 was designed from 9 by replacing the hydrolytically susceptible imine with an olefin ( Fig. 4b ). These changes were not expected to affect MR1 binding directly as neither the C-6 nor C-5 nitrogens of 3c made direct contact with the MR1 protein in the crystal structure [15] ( Fig. 1c ). The conformational agreement of 9 and 10 to 3c was assessed by calculating their energy minimized structures. The iminocarbonyl and the ribityl moieties of 9 were twisted slightly (=8.6° and ψ =4.0°) due to the additional steric bulk at the C-6 amine ( Fig. 4b, c ). Consistent with this, the distances between the carbonyl carbon and the C-6 amine or the 2′-hydroxyl (d 1 and d 2 , respectively) were slightly elongated compared to 3c ( Fig. 4b, d ). The olefin and ribityl moieties of 10 were significantly more twisted (=−16.8° and ψ =−16.3°) with d 1 and d 2 further elongated. Thus, replacing the N -methylamine of 10 with the smaller methylene group gave a third analogue ( 11 ) ( Fig. 4b ), which was expected to have even greater stability due to the removal of a nucleophile. The energy minimized 11 showed greater conformational similarity to 3c , with the enone, uracil ring and the C-6 carbon essentially coplanar ( Fig. 4b, c ). However, the ribityl chain was more distorted, possibly due to a change in hybridization (N- sp 2 to C- sp 3 ) causing a bond angle decrease ( β =123.6 to 112.8°) at the ribityl-uracil linkage site. To assess their antigenic potencies and stabilities, 9–11 were synthesized ( Fig. 5 ). Compound 9 was synthesized via the addition of N -methylribitylamine 12 to chloronitrouracil 13 to give 14 , followed by nitro reduction (to give 15 ) then condensation with methylglyoxal ( Fig. 5a ). Compound 10 was synthesized by first introducing the enone substituent via a Wittig olefination on 16 (prepared via an ortho -lithiation/formylation sequence), followed by an aza-Michael-type chloride displacement by N -methylribitylamine 12 at the doubly activated C-6 position ( Fig. 5b ). The synthesis of 11 ( Fig. 5c ) was challenging, as there was almost no precedence for the synthesis of delicately functionalized 5,6-dialkyl uracils. Our initial approach of C-6 functionalization by directed ortho -lithiation [37] , [38] was unsuccessful, presumably due to chelation effects from the substrate’s polyoxygenated ribityl chain. Subsequently, we envisaged a construction of the uracil ring from the corresponding ribityl β-ketoester 25 , a key retrosynthetic decision that allowed ribose-derived aldehyde 20 (ref. 39 ) to be elaborated with a stabilized ylide 21 without α-epimerization. In the forward synthesis, aldehyde 20 was alkylated with ylide 17 under neutral conditions to give 22 (83%). Contrary to the reported reactivity of ylide 21 under neutral [40] , [41] or basic [42] conditions, we found that 20 reacted with 21 to give only trace amounts of 24 or led to significant α-epimerization under various conditions. Hydrogenation of 22 gave 23 quantitatively and then α-carboxylation with Mander’s reagent [43] gave β-ketoester 25 (70%). Condensation with thiourea gave thiouracil 26 (quant.) [44] , which was desulfurized unconventionally [45] under basic conditions with 1-butene oxide to yield 27 (84%), preserving the acetonide protecting groups. After investigating reaction conditions on the model compound 6-methyluracil, the methyl vinyl ketone moiety of 29 was installed in one step with alkyne 28 (35%). Finally, deprotection of 29 with 1 M HCl in THF gave 11 (78%). The structures of 9 , 10 and 11 and their synthetic precursors were unambiguously confirmed by HRMS and NMR ( Supplementary Methods and Supplementary Figs 31–58 ). 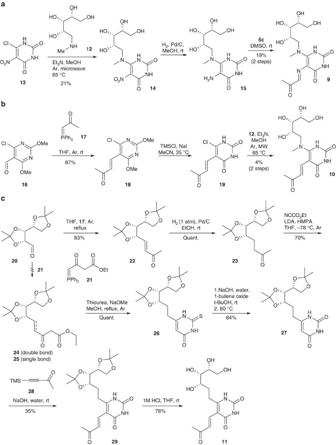Figure 5: Chemical syntheses of uracil-based analogues of 3c as possible antigens. (a) Three step synthesis of9from 5-chloro-6-nitrouracil (13) andN-methylribitylamine (12). (b) Three step synthesis of analogue10from aldehyde16via successive Wittig, nucleophilic demethylation and Michael-type substitution reactions. (c) Seven step synthesis of11from the protected ribose-derived aldehyde20. Successive Wittig and hydrogenation reactions on20, followed by elaboration with Mander’s reagent gave β-ketoester25. Subsequent dehydrative cyclization with thiourea, base mediated desulfurization, ring alkylation and acid mediated global deprotection gave analogue11. Figure 5: Chemical syntheses of uracil-based analogues of 3c as possible antigens. ( a ) Three step synthesis of 9 from 5-chloro-6-nitrouracil ( 13 ) and N -methylribitylamine ( 12 ). ( b ) Three step synthesis of analogue 10 from aldehyde 16 via successive Wittig, nucleophilic demethylation and Michael-type substitution reactions. ( c ) Seven step synthesis of 11 from the protected ribose-derived aldehyde 20 . Successive Wittig and hydrogenation reactions on 20 , followed by elaboration with Mander’s reagent gave β-ketoester 25 . Subsequent dehydrative cyclization with thiourea, base mediated desulfurization, ring alkylation and acid mediated global deprotection gave analogue 11 . Full size image Stability and MAIT cell activation of synthetic analogues The chemical stability and antigenic activities of these analogues were assessed. Despite the additional bulk at the nucleophilic C-6 nitrogen, 9 was less stable than 3c ( Fig. 6a ), cyclizing readily to the corresponding quaternary ammonium species. However, as in 3a , the reduced stability of 9 was consistent with twisting of the iminocarbonyl moiety out of the conjugation plane (=8.6° and ψ =4.0°), likely leading to an increased susceptibility to imine hydration. Although the iminocarbonyl group of enone 10 was even more twisted, it was more stable than 9 as the alkene was more resistant to hydration. Nonetheless, it still degraded to give the corresponding cyclic quaternary ammonium species. Finally, 11 was completely water stable with no degradation observed over 5 days (PBS buffer, pH=7.4, 37 °C). 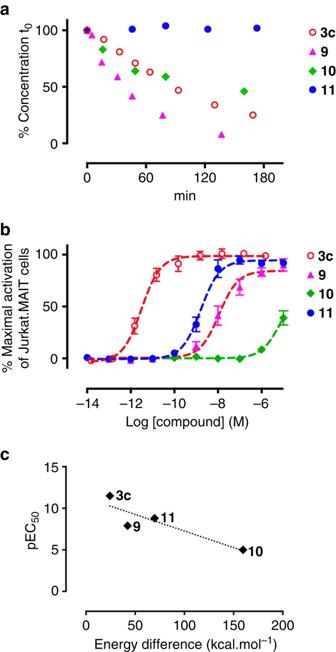Figure 6: Stability and MAIT cell activation of 9, 10 and 11. (a) The aqueous stability of3cand9–11measured by LCMS as a percentage of initial concentration (0.065 mM) over time (37 °C, PBS buffer pH 7.4). (b) MAIT cell activation. Data represent mean±s.e.m. (n=3). (c) Plot of antigen potency (pEC50) versus calculated energy difference between the energy minimized conformers and postulated bioactive conformers of3cand9–11. The biologically active conformers of9–11were created by making the necessary atom connectivity changes to the antigen conformer present in the MR1-3c-TCR crystal structure. Figure 6: Stability and MAIT cell activation of 9, 10 and 11. ( a ) The aqueous stability of 3c and 9 – 11 measured by LCMS as a percentage of initial concentration (0.065 mM) over time (37 °C, PBS buffer pH 7.4). ( b ) MAIT cell activation. Data represent mean±s.e.m. ( n =3). ( c ) Plot of antigen potency (pEC 50 ) versus calculated energy difference between the energy minimized conformers and postulated bioactive conformers of 3c and 9 – 11 . The biologically active conformers of 9 – 11 were created by making the necessary atom connectivity changes to the antigen conformer present in the MR1- 3c -TCR crystal structure. Full size image The antigenic activity of 9 (EC 50 =14±14 nM) was reduced by four orders of magnitude compared to its parent imine 3c , while the more stable enone analogues 10 and 11 exhibited disparate potencies of >10 μM and 1.6 nM, respectively ( Fig. 6b ). These relative potencies were consistent with the hypothesis that a better conformational match to 3c , especially with respect to the dihedral angle ψ , would result in greater antigenic potency ( Fig. 4c ). To support this idea further, the overall conformational distortion of the ligands was quantitatively evaluated, reasoning that the energies expended by 9 – 11 to adopt the ideal bioactive conformation would be related to their antigenic activities. Thus, 9 – 11 were modelled by making the necessary atom connectivity changes to the 3c conformer bound in the MR1- 3c -TCR crystal structure. The energies of these ‘bioactive’ conformers and the energy-minimized conformers were then calculated using Gaussian. Their differences inversely correlated with their activity (pEC 50 ), supporting the conformational matching hypothesis ( Fig. 6c ). Together, 9 – 11 provide an important base for the delineation of further structure-activity relationships to optimize these antigens and to clarify the molecular determinants of MR1 binding versus MAIT cell activation. Functional profiling of analogue 11 To demonstrate the utility of analogue 11 in MAIT cell-related immunological studies, we performed in vitro and in vivo functional assays. We have previously shown upregulation of MR1 surface expression for 3c and also for the MAIT-non-stimulatory MR1 ligand acetyl-6-formylpterin (Ac-6-FP, 30 ) [21] , [46] . Here we incubated C1R.MR1 cells with a range of concentrations of 3c , 9 – 11 or 30 over a 24 h time course and detected MR1 expression by staining with the monoclonal antibody 26.5 ( 3c , 11 and 30 shown in Fig. 7a ; all compounds and dose titration of 3c and 11 shown in Supplementary Fig. 9 ). Compounds 3c and 11 showed comparable early upregulation of MR1, but the upregulation caused by 3c peaked at 4 h then reduced, consistent with turnover of MR1 in the cells [46] and instability of 3c in aqueous solution. In contrast, MR1 surface expression continued to increase over 24 h in the presence of 11 to a similar level as induced by 30 (ref. 46 ), consistent with 11 being chemically more stable in water than 3c . 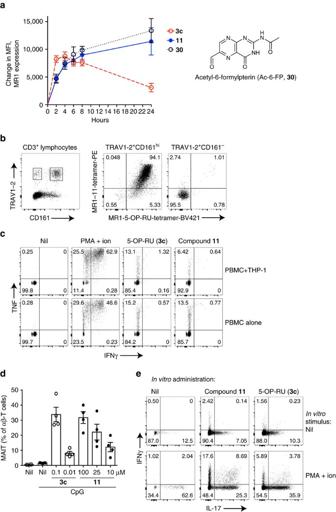Figure 7: Analogue 11 is functionally similar to 5-OP-RU (3c). (a) Upregulation of surface expression of MR1 on C1R.MR1 cells at indicated time points with 10 μM 5-OP-RU3c, compound11or Ac-6-FP (30, structure shown at right). Mean±s.e.m. from three independent experiments (for analogues9and10, and concentration-response curves of 5-OP-RU3cand11at defined time points seeSupplementary Fig. 9). (b) Co-staining of human PBMCs with antibodies to CD3, CD161 and TCR TRAV1–2. Gated CD3+lymphocytes are shown from one representative donor from four. Subsequently gated MAIT (TRAV1-2+CD161hiCD3+) cells and conventional T cells expressing TRAV1–2 (TRAV1-2+CD161hiCD3+) were co-stained with MR1 tetramers from11and 5-OP-RU3c. SeeSupplementary Fig. 10for gating strategy. (c) Cytokine profiles after activation of human PBMCs with 5-OP-RU (3c, 1.28 nM) and11(100 μM). SeeSupplementary Fig. 11for gating strategy. (d) MAIT cells (TCRβ+, MR1-3cTet+) as a percentage of αβ-T cells (TCRβ+) isolated from the lungs of mice intranasally inoculated with CpG plus 5-OP-RU3cor11at indicated doses. Day 7 data are shown (Mean±s.e.m.). 4 mice per group. SeeSupplementary Fig. 12for gating strategy. (e) Cytokine production by MAIT cells harvested from lungs (day 7) of mice inoculated with CpG (day 0) plus 5-OP-RU3c(1 μM) or11(100 μM) four times on day 0, 1, 2 and 4, detected by intracellular cytokine staining either with or without further stimulation with PMA+ionomycin. One representative mouse (from 4) per group is shown. Experiments were performed twice. SeeSupplementary Fig. 12for gating strategy. Figure 7: Analogue 11 is functionally similar to 5-OP-RU (3c). ( a ) Upregulation of surface expression of MR1 on C1R.MR1 cells at indicated time points with 10 μM 5-OP-RU 3c , compound 11 or Ac-6-FP ( 30 , structure shown at right). Mean±s.e.m. from three independent experiments (for analogues 9 and 10 , and concentration-response curves of 5-OP-RU 3c and 11 at defined time points see Supplementary Fig. 9 ). ( b ) Co-staining of human PBMCs with antibodies to CD3, CD161 and TCR TRAV1–2. Gated CD3 + lymphocytes are shown from one representative donor from four. Subsequently gated MAIT (TRAV1-2 + CD161 hi CD3 + ) cells and conventional T cells expressing TRAV1–2 (TRAV1-2 + CD161 hi CD3 + ) were co-stained with MR1 tetramers from 11 and 5-OP-RU 3c . See Supplementary Fig. 10 for gating strategy. ( c ) Cytokine profiles after activation of human PBMCs with 5-OP-RU ( 3c , 1.28 nM) and 11 (100 μM). See Supplementary Fig. 11 for gating strategy. ( d ) MAIT cells (TCRβ + , MR1- 3c Tet + ) as a percentage of αβ-T cells (TCRβ + ) isolated from the lungs of mice intranasally inoculated with CpG plus 5-OP-RU 3c or 11 at indicated doses. Day 7 data are shown (Mean±s.e.m.). 4 mice per group. See Supplementary Fig. 12 for gating strategy. ( e ) Cytokine production by MAIT cells harvested from lungs (day 7) of mice inoculated with CpG (day 0) plus 5-OP-RU 3c (1 μM) or 11 (100 μM) four times on day 0, 1, 2 and 4, detected by intracellular cytokine staining either with or without further stimulation with PMA+ionomycin. One representative mouse (from 4) per group is shown. Experiments were performed twice. See Supplementary Fig. 12 for gating strategy. Full size image Next, we examined whether 11 was capable of refolding MR1 for the generation of tetramer reagents. Indeed, human MR1 was readily refolded in the presence of 11 (not shown) and tetramers were generated in parallel to 3c (that is, MR1-5-OP-RU tetramers [15] , [23] ). When used to detect cells within human peripheral blood mononuclear cells (PBMCs) from four healthy blood donors, >94% of TCR TRAV1-2 + CD161 hi CD3 + cells (MAIT cells) co-stained with both tetramers, but no distinct staining was observed for conventional T cells expressing TRAV1-2 ( Fig. 7b ). To assess the ability of 11 to activate MAIT cells, human PBMCs were cultured alone, or with THP-1 cells, in the presence of the compounds, and cytokine production assessed by intracellular cytokine staining. Similar to 3c , 11 stimulated the production of interferon-γ (IFNγ) and tumour necrosis factor (TNF) by human MAIT cells ( Fig. 7c ), indicating that it is functionally comparable to 3c . Finally, we utilized our established mouse model [47] to examine the MAIT cell response to analogue 11 in vivo . In this model, we previously showed that accumulation of MAIT cells occurs in the lungs after intranasal administration of 3c and a co-stimulant, such as Toll-like receptor (TLR) agonists. Thus, we used TLR agonist CpG oligodeoxynucleotides with either 3c or 11 at a range of doses. Both compounds were capable of causing MAIT cell accumulation in the lungs ( Fig. 7d ), albeit with different efficiencies. Thus, 11 has the same functional profile as 3c in both in vitro and in vivo assays examined to date. MAIT cells are an abundant population of innate-like T cells recognized relatively recently and considered to be involved in many immunological and pathological processes [9] , [48] , [49] , [50] . The identity of the natural antigens was elusive until recently, when we discovered that they were uracil-based imines 3 , formed by a Schiff base condensation between bacterial riboflavin biosynthetic intermediate 1 and the α-dicarbonyl glycolysis metabolites 5 (ref. 15 ). Unfortunately, antigens 3 are very unstable in water, necessitating the development of a practical synthesis in order to more effectively investigate their immunology and pharmacology. We found that although compounds 3a-c form only transiently and in small quantities during the reaction between 1 and 5 in water, they were formed exclusively in high yield as long-lived kinetically stable products in DMSO. Importantly, when 3 was isolated from DMSO, it degraded to 4 much more slowly in water than from mixtures of 1 and 5 in water under the same conditions, suggesting a mechanism involving direct conversion of 6 to 4 with very little formation of the immunologically active 3 in water. Taken together, the superior preparation of 5-OP-RU 3c in DMSO under kinetic control can dramatically improve its utility as an immunological reagent compared to our previously reported aqueous-based preparation ( Fig. 3b, c ). In addition, this study rationalizes mechanistically and demonstrates experimentally the different aqueous stabilities and potencies (EC 50 510 and 1.6 pM, 3b and 3c respectively) of these unstable α-iminocarbonyl compounds as MAIT cell antigens. Compounds 9–11 were synthesized as analogues of 3c in attempts to improve antigen stability, with 11 shown to be the most potent analogue that was completely stable in water. Despite the chemical and structural similarities of 3c and 11 , their different potencies suggest a very specific conformational requirement for antigen recognition of the MR1-TCR complex. Nevertheless, since 11 shows a similar functional profile to 3c in vitro and in vivo , is indefinitely stable in water and easier to handle, it is a potentially useful new reagent for the study of MAIT cells. Furthermore, this study has provided conformational insights for rational design of new MAIT cell antigens and lays the foundation for a better understanding of MAIT cell recognition and activation in immunological responses. General experimental methods for NMR, HPLC and LCMS for monitoring kinetics of formation and stability in aqueous media, and MAIT cell activation assay were conducted as described previously [15] , [17] . Materials Glyoxal, methylglyoxal (both as 40% solutions in water), and butane-2,3-dione (neat) were purchased from Sigma-Aldrich. 5-Amino-6-D-ribitylaminouracil degrades oxidatively in air [31] , [51] , so it was freshly generated under argon in the dark by reduction with sodium dithionite (3 eq) of the corresponding 5-nitroso-6- D -ribitylaminouracil precursor, prepared following a literature procedure [26] with modifications ( Supplementary Information ). Methylglyoxal (40% solution in water) degrades with prolonged storage; to minimize this, new commercial samples were aliquoted and stored at −80 °C. Synthesis and characterization of α-carbonyl imines 3a-c A solution of freshly prepared amine 1 was adjusted to pH 7.0 using 1 M NaOH and lyophilized. The powdered 1 (70 mg, containing sodium sulfate from its preparation) was suspended in DMSO- d 6 (1 g) under argon, and then mixed at rt for 1 min. The mixture was filtered through a HPLC syringe filter to remove salts, degassed in vacuo , purged with argon, and transferred to an NMR tube prefilled with argon. The concentration was determined by PULCON NMR spectroscopy (typically 50 mM, NMR spectra in Supplementary Data 1 ) [52] . Glyoxal (2.0 equivalents), methylglyoxal (1.1 equivalent) or butane-2,3-dione (2.0 equivalents) was added, and the reaction monitored by 1 H NMR. Within 1 h, the reaction was observed clearly and the various unstable α-carbonyl imines 3a and 3b were characterized by 1D and 2D NMR ( Supplementary Figs 15–21 ). In the case of compound 3c , the reaction was allowed to stand at room temperature for 48–72 h to reach completion. The solvent was removed in vacuo at room temperature (4 h) with magnetic stirring. The residue was dissolved in 5 ml of 20 mM pH 5.4 aqueous NH 4 OAc and then immediately purified using a Shimadzu preparative HPLC system equipped with a Phenomenex Luna 10 micron C18 250 × 21.2 mm column (P/No 00G-4253-PO-AX) and a SPD-M20A diode array detector (monitored at wavelength λ365 nm). Flow rate was 20 ml min −1 with linear gradient: 100% solvent A to 100% solvent B over 30 min where solvent A was 20 mM ammonium acetate pH 5.4 in H 2 O and solvent B was 20 mM ammonium acetate pH 5.4 in MeCN-H 2 O (80:20, v/v). Immediately after the collection of the product peak (9.1 min), the pH of the fraction was adjusted accurately to 8.3 with 0.05% w/w ammonia aqueous solution. The solution was frozen immediately (dry ice/acetone bath) and lyophilized in an acid-free environment. The resultant light purple material was redissolved in milliQ water, then immediately frozen and re-lyophilized. The product was obtained as a yellow powder (31% yield; NMR spectra in Supplementary Figs 20–21 ). 5-(1-Methyl-2-oxopropylideneamino)-6-(1- D -ribitylamino)uracil ( 3a ). 1 H NMR (600 MHz, DMSO- d 6 , key signals only): δ 1.83 (s, 3H, N=CMe), 2.40 (s, 3H, MeCO); 13 C NMR (150 MHz, DMSO- d 6 ): δ 17.2 (N=C Me ), 24.9 ( Me CO), 159.8 (N=C), 199.7 (C=O); HRMS ( m / z ): [M] − calcd. for C 13 H 19 N 4 O 7 , 343.1259; found, 343.1250. 5-(2-Oxoethylideneamino)-6-(1- D -ribitylaminouracil ( 3b ): 1 H NMR (600 MHz, DMSO- d 6 , key signals only): δ 8.83 (d, J =8.0 Hz, 1H, N=CH), 9.41 (d, J =8.1 Hz, 1H, CHO); 13 C NMR (150 MHz, DMSO- d 6 ): δ 142.0 (N=C), 194.5 (CH=O); HRMS ( m / z ): [M] − calcd. for C 11 H 15 N 4 O 7 , 315.0946; found, 315.0944. 5-(2-Oxopropylideneamino)-6-(1-D-ribitylamino)uracil 3c : 1 H NMR (600 MHz, DMSO- d 6 ): δ 2.28 (s, 3H, Me), 3.39–3.43 (m, 2H), 3.47–3.51 (m, 1H), 3.52–3.56 (m, 1H), 3.56–3.61 (m, 2H), 3.73 (m, 1H), 7.43 (br s, 1H), 8.80 (s, 1H, N=CH); 13 C NMR (150 MHz, DMSO- d 6 ): δ 23.5 (Me), 44.1, 63.1, 70.7, 72,8, 72.9, 98.5 (C=N– C ), 142.0 (br, N=C), 152.1 (br), 157.6 (br), 159.1, 200.2 (C=O); HRMS ( m/z ): [M] − calcd. for C 12 H 17 N 4 O 7 , 329.1103; found, 329.1116. Chemical characterization data of compound 11 1 H NMR (600 MHz, 10% D 2 O/H 2 O): δ 1.75–1.81 (m, 1H), 1.92–1.98 (m, 1H), 2.35 (s, 3H), 2.79–2.91 (m, 2H), 3.57–3.61 (m, 2H), 3.66–3.69 (m, 1H), 3.74–3.77 (m, 2H), 7.21 (d, J =16.0 Hz, 1H), 7.52 (d, J =16.0 Hz, 1H); 13 C NMR (150 MHz, 10% D 2 O/H 2 O): δ 27.0, 27.2, 30.1, 62.9, 70.7, 72.4, 74.3, 105.9, 127.8, 136.4, 151.9, 161.3, 165.0, 205.2; HRMS ( m/z ): [M] + calcd. for C 14 H 21 N 2 O 7 , 329.1343; found, 329.1348. Stability of compounds 3a-c and 9–11 in aqueous media Stock solutions of either crude ( 3a , 3b and 9 ) or purified compounds ( 3c, 10 and 11 ) in DMSO- d 6 , with a known concentration calibrated using the PULCON NMR technique [52] , were dissolved in aqueous buffers, such as TBS buffer (10 mM Tris, 150 mM NaCl, pH 8.0), PBS (pH 7.4), MilliQ water (pH 6.8), or aqueous ammonium acetate buffer (20 mM, pH 5.4, 150 mM NaCl). Consumption of 3 was monitored by LCMS. The degradation curves and half-lives under various conditions were summarized in Fig. 6a and in Supplementary Fig. 7 . MAIT reporter cell activation assay MAIT reporter cell activation assays and MR1 upregulation assays were performed by slight modifications to reported methods [17] . Briefly, Jurkat cells transduced with genes encoding a MAIT TCR comprising the TRAV1-2-TRAJ33 invariant α chain, and a TRBV6-1 β chain, were tested for activation by co-incubation with compounds and C1R antigen-presenting cells expressing MR1 (CIR.MR1) for 16 h or over a time course as indicated. Cells were subsequently stained with PE-Cy7-conjugated anti-CD3 (UCHT1, eBioscience, 1:300), and APC-conjugated anti-CD69 (BD, 1:25) antibodies as well as biotinylated anti-MR1 mAb 26.5, a gift from Dr Ted Hansen, Washington University School of Medicine, St Louis, MO [53] , followed by Streptavidin-PE (BD, 1:1,000), before analysis by on a FACS CantoII (BD) flow cytometer. Activation of Jurkat.MAIT was measured by an increase in surface CD69 expression. MR1 expression was detected on gated C1R.MR1 cells in the same assay. Generation of MR1–11 and MR1-5-OP-RU tetramers MR1 refolding was performed by slight modifications to reported methods [17] . Human MR1-5-OP-RU 3c , human MR1–11 tetramers, and mouse MR1-5-OP-RU tetramers were prepared by known methods [15] . Genes encoding soluble human MR1 or human β2m were expressed for 4 h in BL21 E. coli following induction with 1 mM isopropyl β- D -1-thiogalactopyranoside. E. coli were pelleted and resuspended in a buffer containing 50 mM Tris, 25% (w/v) sucrose, 1 mM EDTA, 10 mM DTT pH 8.0. Inclusion body protein was then extracted by lysis of bacteria in a buffer containing 50 mM Tris pH 8.0, 1% (w/v) Triton X-100, 1% (w/v) sodium deoxycholate, 100 mM NaCl, 10 mM DTT, 5 mM MgCl 2 and 1 mg DNaseI per litre of starting culture; and subsequent steps involved homogenization with a polytron homogenizer, centrifugation, and washing inclusion body protein sequentially with firstly a buffer containing 50 mM Tris pH 8.0, 0.5% Triton X-100, 100 mM NaCl, 1 mM EDTA, 1 mM DTT, and secondly a buffer containing 50 mM Tris pH 8.0, 1 mM EDTA, 1 mM DTT. Inclusion body protein was then resuspended in a buffer containing 20 mM Tris pH 8.0, 8 M urea, 0.5 mM EDTA, 1 mM DTT and following centrifugation the supernatant containing solubilized, denatured inclusion body protein was collected and stored at −80 °C. C-terminal cysteine-tagged MR1 and β2m were refolded with ligand essentially as described [15] . Briefly, in order to generate MR1-5-OP-RU and MR1– 11 , 28 mg of MR1 and 14 mg of β2m inclusion body proteins were refolded with 5-A-RU (5.25 μmol) and methylglyoxal (1.77 mmol), or compound 11 (1.92 μmol), respectively. Refolded MR1-Ag was then purified by sequential DEAE (GE Healthcare) anion exchange, S75 16/60 (GE Healthcare) gel filtration, and MonoQ (GE Healthcare) anion exchange chromatography. Cysteine-tagged-MR1-5-OP-RU or MR1– 11 were then reduced with 5 mM DTT for 20 min prior to buffer exchange into PBS using a PD-10 column (GE Healthcare), and biotinylated with Maleimide-PEG2 biotin (Thermoscientific) with a 30:1 molar ratio of biotin:protein at 4 °C for 16 h in the dark. Biotinylated MR1 was subjected to S200 10/300 GL (GE Healthcare) chromatography to remove excess biotin. Biotinylated, MR1-5-OP-RU or MR1–11 monomers were tetramerized with streptavidin conjugated to either PE (SA-PE) or Brilliant Violet 421 (SA-BV) (BD Pharmingen). Tetramer staining of human PBMCs Healthy donor blood packs were obtained through the Australian Red Cross Blood Service after approval from the Melbourne University Human Research Ethics Committee and PBMCs were prepared by separation on Ficoll–Paque Premium (GE Healthcare). Cells were then washed twice prior to resuspension in 10% DMSO in FCS. Prior to use, PBMCs were stored in liquid nitrogen. Approximately 2 × 10 6 cells were stained with human MR1-5-OP-RU tetramer (BV421), human MR1– 11 tetramer (PE) and monoclonal antibodies to CD3 (AlexaFluor700, OKT3, eBioscience, 1:50), CD161 (PE-Cy7, HP-3G10, Biolegend, 1:50) and TRAV1–2 (APC, clone 3C10, Biolegend, 1:50) for 30 min on ice and fixed in 1% paraformaldehyde before acquisition of data on a BD LSR-Fortessa. Data were analyzed using FlowJo software (Tree Star). In vitro PBMC stimulation assay Stimulation of PBMCs was performed essentially as previously described [17] . Briefly, 5 × 10 5 PBMCs were cultured, alone or with 1 × 10 5 THP-1 cells, overnight with or without compounds 3c or 11 at a range of doses or with PMA and ionomycin (5 ng ml −1 and 1 μg ml −1 final concentrations, respectively) as a positive control. BD GolgiStop (1:1,000 dilution) was added after the first hour of stimulation. Cells were stained for surface markers using human MR1-5-OP-RU tetramer (PE, 1:300), and monoclonal antibodies to CD3 (PE-CF594, UCHT1, BD Horizon, 1:50), CD161 (PE-Cy7, HP-3G10, Biolegend, 1:50) for 30 min on ice and fixed in 1% paraformaldehyde before cytokine production by MAIT cells was detected by intracellular cytokine staining with monoclonal antibodies to TNF (APC, MAb11, eBioscience, 1:50) and IFNγ (AlexaFluor700, B27, BD 1:50) in the presence of 0.3% saponin. Data was acquired on a BD LSR-Fortessa and analysed using FlowJo software (Tree Star). In vivo assay Mice were bred and housed at the Biological Research Facility of the Peter Doherty Institute (Melbourne, Victoria, Australia). Male adult (6–10 weeks) C57BL/6 mice were used for all experiments, after approval by the University of Melbourne Animal Ethics Committee. CpG 1688 sequence: 5′-T*C*C*A*T*G*A*C*G*T*T*C*C*T*G*A*T*G*C*T-3′ (*phosphorothioate linkage) nonmethylated cytosine-guanosine oligonucleotides was purchased from Geneworks (Australia). Mice were inoculated with 20 μg CpG once per nares, plus 3c or 11 at indicated doses and MAIT cells were detected from lungs at day 7 as previously described [47] . Cytokine production by isolated MAIT cells was detected by intracellular cytokine staining [47] . Briefly, mice were sacrificed by administration of CO 2 and lungs taken following heart perfusion with 10 ml cold RPMI. To prepare single cell suspensions, lungs were finely chopped with a scalpel blade and treated with 3 mg ml −1 collagenase III (Worthington), 5 μg ml −1 DNAse and 2% FCS in RPMI for 90 min at 37 °C with gentle shaking. Cells were then filtered (70 μM) and washed with PBS/2% FCS. RBCs were lysed with hypotonic buffer TAC (Tris-based Amino Chloride) for 5 min at 37 °C. Approximately 1.5 × 10 6 cells were filtered (40 μm) and used for flow cytometric analysis. Ab against CD19 (1D3, PerCP-Cy 5.5, 1:200), CD45.2 (104, FITC, 1:200), IFNγ (XMG1.2, PE-Cy7, 1:400), TCRβ (H57–597, APC or FITC, 1:200) and IL-17A (TC11-18H10, PE, 1:200) were purchased from BD. To block non-specific staining, cells were incubated with MR1-6FP tetramer and anti-Fc receptor (2.4G2) for 15 min at room temperature, then incubated at room temperature with antibody/tetramer cocktails in PBS/2% FCS. 7-AAD (5 μl per sample) was added for the last 10 min. Cells were fixed with 1% PFA prior to analysis on LSR Fortessa (BD Bioscience) flow cytometer. Data analysis was performed with FlowJo software. For intracellular cytokine staining (ICS), Golgi plug (BD Biosciences) was used during all processing steps. Cells stimulated with PMA/Ionomycin (20 ng ml −1 , 1 μg ml −1 respectively) for 3 h at 37 °C were included as positive controls. FVD (eBioscience) were added for 30 min at 4 °C before surface staining. Surface staining was performed at 37 °C and cells stained for intracellular cytokines using the BD Fixation/Permeabilisation kit or transcription factors using the transcription buffer staining set (eBioscience) according to the manufacturers’ instructions. Data availability The authors declare that the data supporting the findings of this study are available within the paper and its Supplementary Information files . FIDs of the NMR spectra are available from the authors upon request. How to cite this article: Mak, J. Y. W. et al . Stabilizing short-lived Schiff base derivatives of 5-aminouracils that activate mucosal-associated invariant T cells. Nat. Commun. 8, 14599 doi: 10.1038/ncomms14599 (2017). Publisher’s note: Springer Nature remains neutral with regard to jurisdictional claims in published maps and institutional affiliations.